ZBTB20 regulates nociception and pain sensation by modulating TRP channel expression in nociceptive sensory neurons In mammals, pain sensation is initiated by the detection of noxious stimuli through specialized transduction ion channels and receptors in nociceptive sensory neurons. Transient receptor potential (TRP) channels are the key sensory transducers that confer nociceptors distinct sensory modalities. However, the regulatory mechanisms about their expression are poorly defined. Here we show that the zinc-finger protein ZBTB20 regulates TRP channels expression in nociceptors. ZBTB20 is highly expressed in nociceptive sensory neurons of dorsal root ganglia. Disruption of ZBTB20 in nociceptors led to a marked decrease in the expression levels of TRPV1, TRPA1 and TRPM8 and the response of calcium flux and whole-cell currents evoked by their respective specific agonists. Phenotypically, the mice lacking ZBTB20 specifically in nociceptors showed a defect in nociception and pain sensation in response to thermal, mechanical and inflammatory stimulation. Our findings point to ZBTB20 as a critical regulator of nociception and pain sensation by modulating TRP channels expression in nociceptors. In mammals, the perception of pain is initiated by the detection of noxious thermal, mechanical and chemical stimuli through the peripheral nerve fibres from a specialized subpopulation of primary sensory neurons, called nociceptors [1] , [2] . Nociceptors are highly diversified with different sensory modalities. There are two major subsets of small DRG neurons. One subset is peptidergic, which expresses receptor tyrosine kinase TrkA, the receptor of nerve growth factor, and synthesizes neuropeptides like calcitonin gene-related peptide (CGRP) and substance P. The other is nonpeptidergic, which expresses the c-Ret neurotrophin receptor, and responds to glial-derived neurotrophic factor, as well as neurturin and artemin. Most c-Ret-positive neurons are capable of binding the isolectin IB4 and express Mas-related G-protein-coupled receptors (Mrgpr) [3] , and specific purinergic receptor subtypes, notably P2X3. Nociceptors are equipped with a diverse array of ion channels that act as sensory transducer, each specialized to only respond to particular stimuli and initiate electrical activity. Among them, transient receptor potential (TRP) ion channels have emerged as a major sensory transducer family, with many members involved specifically in generating thermally and chemically evoked pain sensations [4] . For example, TRPV1, TRPV2, TRPV3 and TRPV4 act as thermal receptors [5] . TRPV1 and TRPV2 channels display a temperature activation threshold of 43 and 52 °C, respectively, whereas TRPV3 and TRPV4 are activated between 25 and 35 °C (ref. 2 ). TRPV1 marks a population of unmyelinated, slowly conducting neurons (C-fibres) that express the neuropeptides substance P, neurokinin A and CGRP and constitute ~30–50% of all somatosensory neurons within rodent sensory ganglia [6] . As an endogenous transducer of noxious heat, TRPV1 is essential for selective modalities of pain sensation and tissue injury-induced thermal hyperalgesia [7] . TRPV2 is expressed in a subpopulation of Aδ neurons that respond to high-threshold noxious heat. Actually, TRPV3 and TRPV4 belong to ‘innocuous’ warm detectors [8] , [9] . Furthermore, TRPM8 and TRPA1 putatively act as cold pain receptors [10] , [11] . TRPM8 is robustly expressed by ~15% of all somatosensory neurons encompassing mostly small-diameter, unmyelinated C-fibres, as well as a minor cohort of lightly myelinated Aδ fibres. TRPM8 is activated at cool temperatures (~26 °C) and by the cooling compound menthol [10] , [12] . Mouse knockout studies have revealed that TRPM8 is required for cold sensation over a broad range of innocuous and noxious cold temperatures [13] , [14] , [15] . TRPA1 is largely restricted to TRPV1-positive neurons [16] , and acts as a major sensor for noxious cold and plays an important role in chemonociception by serving as a detector of chemical irritants that elicit acute and inflammatory pain [6] , [11] . Remarkably, many TRP channels are generally expressed by nociceptors in a partially overlapping or mutually exclusive fashion. For example, TRPV1 and TRPM8 segregate into different classes of nociceptors in mouse DRG [17] , [18] . Therefore, nociceptors can also be distinguished according to their differential expression of ion channels that confer sensitivity to heat (TRPV1), cold (TRPM8) and a host of chemical irritants (TRPA1) (ref. 19 ). Precise regulation of the expression of these ion channels is crucial for their sensory role in nociception. However, the underlying mechanisms are still largely unknown. Several transcription factors have been demonstrated to control the development and differentiation of nociceptive sensory neurons. The neuronal determination gene Neurogenin1 ( Ngn1 ) is required for the formation of most nociceptors [20] . The homeobox gene Brn3a and the zinc-finger gene Klf7 are required for the expression of TrkA and the survival of nociceptors [21] , [22] , [23] . Runx1, a Runt domain transcription factor, controls neuronal diversification within Ngn1 -dependent TrkA + neurons by repressing CGRP expression and coordinates the expression of many ion channels and receptors in nociceptors, including TRP class thermal receptors, Na + -gated, ATP-gated and H + -gated channels, the opioid receptor MOR and Mrgpr [18] , [24] . Furthermore, the transcription factor Tlx3 acts in combination with Runx1 to control the development of a cohort of nociceptors, thermoceptors, and pruriceptors in mice [25] . To date, the transcription factors that specifically regulate the differential expression of nociceptive TRP channels have not been identified. Zinc-finger and BTB domain containing protein 20 (ZBTB20, also known as DPZF, HOF and Zfp288) belongs to a subfamily of zinc-finger proteins containing C2H2 Krüppel-type zinc fingers and BTB/POZ domains [26] , [27] . ZBTB20 is highly expressed in central nervous system and plays a critical role in hippocampal development and function [27] , [28] , [29] , [30] , [31] , but its function in peripheral nervous system is rarely known. In the present study, we found that ZBTB20 was highly expressed in nociceptive sensory neurons in mouse DRG and tissue-specific ablation of ZBTB20 in nociceptors led to a robust decrease both in the expression of TRPV1, TRPM8 and TRPA1 and the pain sensitivity to thermal, mechanical and inflammatory stimuli. These findings point to ZBTB20 as a novel nociceptive regulator through specifically modulating TRP channels expression in DRG. ZBTB20 is highly expressed in nociceptive sensory neurons To characterize the developmental regulation of ZBTB20 expression in nociceptors, we first examined its expression in the developing DRG at different embryonic stages. Immunohistochemical analysis demonstrated that ZBTB20 protein was first detected in the DRG as early as embryonic day 13.5 (E13.5), and was increased by E14.5 ( Supplementary Fig. 1 ). In the DRG of adult mice, double immunostaining showed that ZBTB20 was highly expressed in peripherin-positive small neurons, but was hardly detected in neurofilament (N200)-positive large neurons ( Fig. 1a,b ). To further characterize its expression in nociceptive sensory neurons, we performed double immunostaining of ZBTB20 and Na v 1.8, a sensory neuron-specific voltage-gated sodium channel expressed in >85% of nociceptors [32] , [33] . ZBTB20 protein was detected in the majority (75.2%±3.2%) of Na v 1.8-positive neurons ( Fig. 1c ). These data suggest that ZBTB20 is preferentially expressed in nociceptive sensory neurons, and might be involved in nociception. 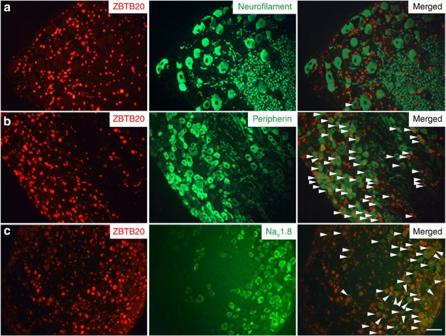Figure 1: ZBTB20 expression in the adult DRG. (a–c) Double immunofluorescent staining showed ZBTB20 expression was undetected in large neurofilament-positive neurons (a), but present in most small peripherin-positive neurons (b) and Nav1.8-positive neurons (c). Double-labelled neurons are indicated by arrowheads. (Scale bar, 50 μm.) Figure 1: ZBTB20 expression in the adult DRG. ( a – c ) Double immunofluorescent staining showed ZBTB20 expression was undetected in large neurofilament-positive neurons ( a ), but present in most small peripherin-positive neurons ( b ) and Na v 1.8-positive neurons ( c ). Double-labelled neurons are indicated by arrowheads. (Scale bar, 50 μm.) Full size image Tissue-specific ablation of ZBTB20 in nociceptors To evaluate the potential role of ZBTB20 in nociceptive neurons, we generated peripheral nociceptor-specific ZBTB20 knockout mice (hereafter referred to as PN-ZB20KO) by crossing ZBTB20 flox mice to Na v 1.8-Cre transgenic mice [34] . This Cre transgenic line has the capacity to mediate Cre/LoxP recombination and gene deletion specifically in nociceptive neurons, starting from as early as E14 as demonstrated by LacZ reporter and X-Gal staining [35] . Efficient deletion of ZBTB20 gene in the DRG of PN-ZB20KO mice was confirmed at the messenger RNA (mRNA) level by real-time RT–PCR and at the protein level by immunoblot analysis with an anti-ZBTB20 antibody 9A10 ( Fig. 2a,b , and Supplementary Fig. 11 ). As expected, the expression of ZBTB20 was unchanged in the spinal cord or brain in PN-ZB20KO mice compared with controls ( Fig. 2a ). Double immunostaining showed that ZBTB20 was only detected in the minority (5.1%±0.3%) of Na v 1.8-positive neurons of PN-ZB20KO mice, which was robustly decreased compared with control mice (75.2±3.2%, P <0.01) ( Fig. 2c ). These results indicated that we successfully generated tissue-specific knockout mice of ZBTB20 in nociceptors. 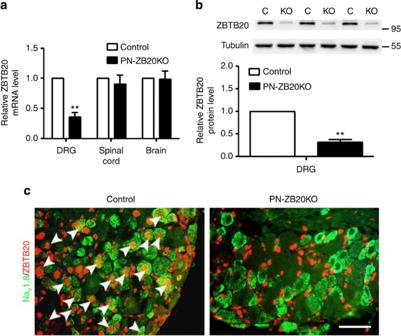Figure 2: Generation of PN-ZB20KO mice. (a) Quantitative RT–PCR analysis for ZBTB20 mRNA in DRG, spinal cord and brain from control and PN-ZB20KO mice. The RT–PCR was performed twice (n=6, **P<0.01 versus control, Student’st-test). (b) Western blot analysis for ZBTB20 expression in DRG from control and PN-ZB20KO mice. C, control. KO:PN-ZB20KO (n=6, **P<0.01 versus control, Student’st-test). Full-size blots are shown inSupplementary Fig. 11. (c) Efficient and specific deletion of ZBTB20 in Nav1.8-positive neurons demonstrated by double immunofluorescence staining of ZTBT20 (red) and Nav1.8 (green). Double-labelled neurons are marked by arrowhead. (Scale bar, 50 μm) Values are the mean±s.e.m. Figure 2: Generation of PN-ZB20KO mice. ( a ) Quantitative RT–PCR analysis for ZBTB20 mRNA in DRG, spinal cord and brain from control and PN-ZB20KO mice. The RT–PCR was performed twice ( n =6, ** P <0.01 versus control, Student’s t -test). ( b ) Western blot analysis for ZBTB20 expression in DRG from control and PN-ZB20KO mice. C, control. KO:PN-ZB20KO ( n =6, ** P <0.01 versus control, Student’s t -test). Full-size blots are shown in Supplementary Fig. 11 . ( c ) Efficient and specific deletion of ZBTB20 in Na v 1.8-positive neurons demonstrated by double immunofluorescence staining of ZTBT20 (red) and Na v 1.8 (green). Double-labelled neurons are marked by arrowhead. (Scale bar, 50 μm) Values are the mean±s.e.m. Full size image Normal morphogenesis of DRG neurons in PN-ZB20KO mice Then we examined whether genetic deletion of ZBTB20 in Na v 1.8-positive neurons could affect the development of DRG neurons. As shown in Supplementary Fig. 2a , the total number of neurons in the lumbar 4 (L4) DRG was similar between adult PN-ZB20KO and control mice. Moreover, percentages of peripherin-positive small neurons (62.7±2.4% in control mice versus 61.3%±2.0% in PN-ZB20KO mice) and neurofilament-positive large neurons (31.2±2.2% in control mice versus 33.2±2.5% in PN-ZB20KO mice) were almost the same as those of controls ( Supplementary Fig. 2b ), showing that the generation of the two major components of DRG neurons is normal in PN-ZB20KO mice. We further investigated two major subsets of small DRG neurons by immunostaining or in situ hybridization. In the DRG sections from L4 of PN-ZB20KO mice, IB4-binding nonpeptidergic neurons (29.6±2.8% in control mice versus 27.7±3.0% in PN-ZB20KO mice) and CGRP-expressing peptidergic neurons (23.2±2.7% in control mice versus 24.4±3.1% in PN-ZB20KO mice) were present at normal levels ( Fig. 3a ). Similarly, percentages of TrkA-positive neurons (30.2±3.1% in control mice versus 28.8±2.9% in PN-ZB20KO mice) and Ret-positive neurons (65.4±5.2% in control mice versus 67.7±5.6% in PN-ZB20KO mice) were not significantly different between the two groups ( Fig. 3b ). These data indicated that morphogenesis of DRG neurons was largely normal in PN-ZB20KO mice. 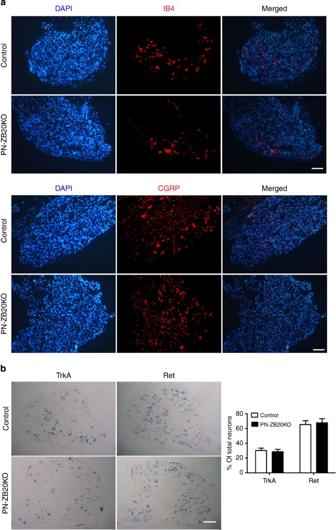Figure 3: Normal morphogenesis of DRG neurons in PN-ZB20KO mice. (a) DRG sections were labelled with lectin IB4-biotin or anti-CGRP antibody. IB4-binding nonpeptidergic neurons and CGRP-expressing peptidergic neurons were present at normal levels in DRG of PN-ZB20KO mice (Scale bar, 100 μm). (b)In situhybridization performed with TrkA and Ret probes, and the numbers of neurons that express these markers were not significantly different between the two groups (Scale bar, 100 μm). About 9–12 DRG sections per animal (three animals of each genotype) were analysed. Data were analysed by Student’st-test. Values are the mean±s.e.m. Figure 3: Normal morphogenesis of DRG neurons in PN-ZB20KO mice. ( a ) DRG sections were labelled with lectin IB4-biotin or anti-CGRP antibody. IB4-binding nonpeptidergic neurons and CGRP-expressing peptidergic neurons were present at normal levels in DRG of PN-ZB20KO mice (Scale bar, 100 μm). ( b ) In situ hybridization performed with TrkA and Ret probes, and the numbers of neurons that express these markers were not significantly different between the two groups (Scale bar, 100 μm). About 9–12 DRG sections per animal (three animals of each genotype) were analysed. Data were analysed by Student’s t -test. Values are the mean±s.e.m. Full size image The gene deletion mediated by Na v 1.8-Cre occurs at E14 in small-diameter neurons of DRG [35] , a little lagging behind their early expression of ZBTB20 at E13.5, thus we reasoned that PN-ZB20KO mice might not reflect the function of ZBTB20 in the early stage of neuronal morphogenesis in DRG. To exclude this possibility, we generated another conditional knockout mice lacking ZBTB20 in nervous system (hereafter NS-ZB20KO) using the Nestin-Cre transgenic mice, which mediates conditional gene deletion by E11 (ref. 36 ). In the L4 DRG of adult NS-ZB20KO mice, the total number of neurons (4,876±182 in control mice versus 4,754±193 in NS-ZB20KO mice), IB4-binding nonpeptidergic neurons (27.4%±2.5% in control mice versus 30.1±3.2% in NS-ZB20KO mice) and CGRP-expressing peptidergic neurons (24.4±2.8% in control mice versus 22.1±2.6% in NS-ZB20KO mice) were present at normal levels ( Supplementary Figs 3 and 4 ). Furthermore, percentages of TrkA-positive neurons (28.4±2.0% in control mice versus 30.5±2.3% in NS-ZB20KO mice) and Ret-positive neurons (66.4±4.3% in control mice versus 65.3±4.5% in NS-ZB20KO mice) were almost the same as those of controls ( Supplementary Fig. 5 ). Taken together, our results suggest ZBTB20 is dispensable for the morphogenesis of DRG neurons. Altered TRP channels expression in DRG of PN-ZB20KO mice The expression of high-threshold ion channels defines the specialized peripheral-receptive properties of nociceptor subclasses. To determine if ZBTB20 is required for the specification of different transduction phenotypes, we analysed the expression of nociceptive ion channels and sensory receptors in PN-ZB20KO. In situ hybridization showed that the percentage of TRPV1-positive neurons in lumbar DRG was decreased from 34.2±4.1% in control mice to 17.5±2.8% in PN-ZB20KO mice, and the percentage of TRPA1-positive neurons also decreased from 30.5±3.4% to 14.2±1.9% ( Fig. 4 ). The percentage of TRPM8-positive neurons was not significantly affected in the DRG of PN-ZB20KO mice (13.8±1.7% versus 12.6±1.5%), but their signal intensity of TRPM8 mRNA was significantly decreased compared with control. Other nociceptive ion channels and sensory receptors, including TRPV2, P2X3, Na v 1.7, Na v 1.8, Na v 1.9 and Mrgpr members (Mrgprd, Mrgpr4 and Mrgpr5), did not show significant difference by in situ hybridization between control and PN-ZB20KO mice ( Fig. 4 , and Supplementary Fig. 6 ). Furthermore, immunostaining also demonstrated that ZBTB20 deficiency led to a dramatic decrease in the percentage of both TRPV1 neurons and TRPA1 neurons in adult DRG ( Fig. 5a,b ). Despite the unaffected percentage of total TRPM8 neurons in PN-ZB20KO DRG, their percentage of TRPM8 high-positive neurons, together with TRPV1 high-positive neurons, was robustly reduced compared with control group. Western blot analysis showed that TRPV1, TRPA1 and TRPM8 protein levels were significantly decreased in the DRG of PN-ZB20KO mice ( Fig. 5c , and Supplementary Fig. 12 ). Despite these alterations of these TRP channels, the expression of Runx1, which regulates a large cohort of ion channels and receptors [18] , was not affected in the DRG neurons by the disruption of ZBTB20 ( Fig. 4 ). Taken together, these results suggest that ZBTB20 may regulate a subset of TRP channels in nociceptors in a Runx1-independent manner. Double immunohistochemical staining revealed that ZBTB20 protein was detected in the majority of adult TRPV1-positive, TRPA1-positive or TRPM8-positive DRG neurons in wild-type mice ( Fig. 5d ), suggesting that ZBTB20 may regulate the expression of TRPV1, TRPA1 and TRPM8 in a cell-autonomous manner. 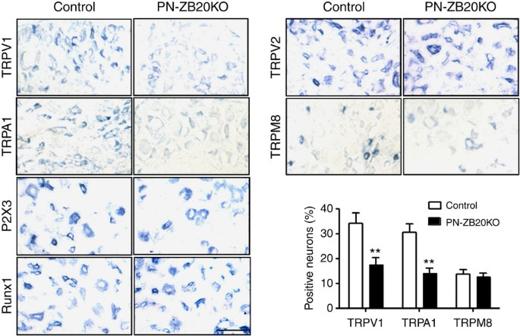Figure 4: TRP channel mRNA expression is decreased in DRG neurons from PN-ZB20KO mice. In situhybridization performed with TRPV1, TRPA1, TRPM8 or other probes (Scale bar, 50 μm). The percentage of TRPV1-positive or TRPA1-positive neurons is significantly decreased (**P<0.01 versus control, Student’st-test). Although the percentage of TRPM8-positive neurons was not significantly changed in the DRG of PN-ZB20KO mice, the signal intensity was significantly weaker than control. About 9–12 DRG sections per animal (three animals of each genotype) were analysed **P<0.01 versus control. Values are the mean±s.e.m. Figure 4: TRP channel mRNA expression is decreased in DRG neurons from PN-ZB20KO mice. In situ hybridization performed with TRPV1, TRPA1, TRPM8 or other probes (Scale bar, 50 μm). The percentage of TRPV1-positive or TRPA1-positive neurons is significantly decreased (** P <0.01 versus control, Student’s t -test). Although the percentage of TRPM8-positive neurons was not significantly changed in the DRG of PN-ZB20KO mice, the signal intensity was significantly weaker than control. About 9–12 DRG sections per animal (three animals of each genotype) were analysed ** P <0.01 versus control. Values are the mean±s.e.m. 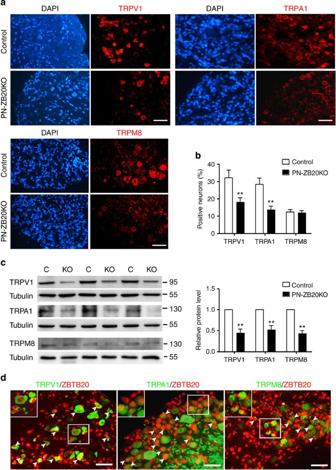Figure 5: Decreased expression of pain-associated channels or receptors in the DRG of PN-ZB20KO mice. (a) DRG sections of PN-ZB20KO and control mice were labelled with anti-TRPV1, anti-TRPA1 or anti-TRPM8 antibodies. (b) The proportion of TRPV1-expressing or TRPA1-expressing neurons was significantly decreased in PN-ZB20KO mice (**P<0.01 versus control, Student’st-test). Although the percentage of TRPM8-positive neurons was not significantly changed in the DRG of PN-ZB20KO mice, the fluorescence intensity was significantly weaker than control. Four to seven independent L4 DRG were used for each counting. (Scale bar, 50 μm). (c) Western blot analysis showed that TRPV1, TRPA1 and TRPM8 protein levels were significantly decreased in the DRG of PN-ZB20KO mice. Full-size blots are shown inSupplementary Fig. 12. C, control mice. KO:PN-ZB20KO mice (n=6; **P<0.01 versus control, Student’st-test). (d) Double labelling of ZBTB20 protein (red) and TRPV1 (green), TRPA1 (green) or TRPM8 (green) on adult wild-type DRG sections. Note that ZBTB20 was expressed in the majority of neurons expressing TRPV1, TRPA1 or TRPM8 (green). Double-labelled neurons are marked by arrowhead. (Scale bar, 50 μm). Values are the mean±s.e.m. Full size image Figure 5: Decreased expression of pain-associated channels or receptors in the DRG of PN-ZB20KO mice. ( a ) DRG sections of PN-ZB20KO and control mice were labelled with anti-TRPV1, anti-TRPA1 or anti-TRPM8 antibodies. ( b ) The proportion of TRPV1-expressing or TRPA1-expressing neurons was significantly decreased in PN-ZB20KO mice (** P <0.01 versus control, Student’s t -test). Although the percentage of TRPM8-positive neurons was not significantly changed in the DRG of PN-ZB20KO mice, the fluorescence intensity was significantly weaker than control. Four to seven independent L4 DRG were used for each counting. (Scale bar, 50 μm). ( c ) Western blot analysis showed that TRPV1, TRPA1 and TRPM8 protein levels were significantly decreased in the DRG of PN-ZB20KO mice. Full-size blots are shown in Supplementary Fig. 12 . C, control mice. KO:PN-ZB20KO mice ( n =6; ** P <0.01 versus control, Student’s t -test). ( d ) Double labelling of ZBTB20 protein (red) and TRPV1 (green), TRPA1 (green) or TRPM8 (green) on adult wild-type DRG sections. Note that ZBTB20 was expressed in the majority of neurons expressing TRPV1, TRPA1 or TRPM8 (green). Double-labelled neurons are marked by arrowhead. (Scale bar, 50 μm). Values are the mean±s.e.m. Full size image To explore the mechanisms by which ZBTB20 regulates the expression of these TRP genes, we examined the association of ZBTB20 protein with their promoters individually by chromatin immunoprecipitation (ChIP). ChIP assays were performed with antibodies against ZBTB20, acetylated histone 3 (positive control) or control immunoglobulin G as negative control of chromatin recovery, and the recovered chromatin DNA was subjected to PCR analysis. As shown in Supplementary Fig. 7 , ZBTB20 did not bind to the promoters of TRPV1 , TRPA1 or TRPM8 genes. These results suggest that ZBTB20 most likely regulates the expression of these channels by indirect mechanisms. Decreased calcium influx of TRP channels in PN-ZB20KO DRG To assess the electrophysiological properties of TRPV1, TRPA1 and TRPM8 channels in PN-ZB20KO nociceptors, we first measured calcium fluxes of primary adult DRG neurons in response to the stimulation of 1 μM capsaicin (an agonist of TRPV1) [7] , 100 μM mustard oil (MO, an agonist of TRPA1) [11] and 250 μM menthol (an agonist of TRPM8) (ref. 14 ), respectively. About 42% (76/182) of recorded control DRG neurons showed capsaicin-evoked increase of [Ca 2+ ] i , while there was only 21% (39/186) in PN-ZB20KO DRG neurons ( Fig. 6a ). In the responded DRG neurons, the amplitude of the capsaicin-evoked responses was diminished by about 65% in PN-ZB20KO mice compared with control counterpart ( Fig. 6b,c ). We observed similar phenomenon in PN-ZB20KO DRG neurons when neurons were stimulated by 100 μM MO ( Fig. 6d–f ). Furthermore, about 8.6% (23/266) of recorded DRG neurons showed menthol-evoked increase of [Ca 2+ ] i in control mice. However, it was only 2.7% (7/258) in PN-ZB20KO mice ( Fig. 6g ). In the responded DRG neurons, the amplitude of the menthol-evoked responses was diminished by about 55% in PN-ZB20KO mice compared with that of control neurons ( Fig. 6h,i ). 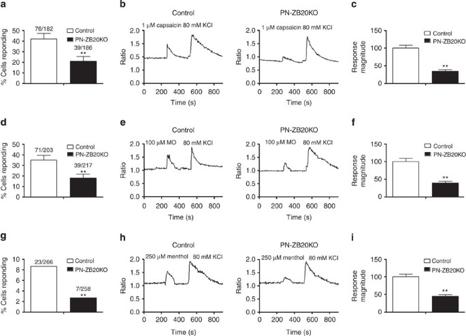Figure 6: TRP channels agonist-evoked calcium flux responsiveness were impaired in DRG neurons from PN-ZB20KO mice. Primary DRG neurons were isolated from adult control and PN-ZB20KO mice, stimulated with 1 μM capsaicin (TRPV1 agonist), 100 μM MO (TRPA1 agonist) or 250 μM menthol (TRPM8 agonist) and their calcium flux was monitored. (a) Capsaicin-responsive neurons were significantly decreased in the DRG from PN-ZB20KO mice. (b) Representative traces of Ca2+transients evoked by 1 μM capsaicin in DRG neurons of control and PN-ZB20KO mice. A quantity of 80 mM KCl was used to check the viability of the neurons at the end of the experiment. (c) The response magnitude was significantly lower in the remaining capsaicin-responsive neurons from PN-ZB20KO DRG than their control counterpart. (d) MO-responsive neurons were significantly decreased in the DRG from PN-ZB20KO mice. (e) Representative traces of Ca2+transients evoked by 100 μM MO in DRG neurons of control and PN-ZB20KO mice. A quantity of 80 mM KCl was used to check the viability of the neurons at the end of the experiment. (f) The response magnitude was significantly lower in the remaining MO-responsive neurons from PN-ZB20KO DRG than their control counterpart. (g) In neurons from PN-ZB20KO mice, the percentage of menthol-responsive neurons was significantly less than those seen in neurons from control mice. (h) Representative traces of Ca2+transients evoked by 250 μM menthol in DRG neurons of control and PN-ZB20KO mice. A quantity of 80 mM KCl was used to check the viability of the neurons at the end of the experiment. (i) In neurons from PN-ZB20KO mice, the magnitude of remaining responses to menthol was significantly less than those seen in neurons from control mice. The numbers of responsive and total neurons (pooled from all experiments for each genotype) are indicated in (a,d,j). (a,c,d,f,g,i) Data were analysed by Student’st-test. **P<0.01 versus control. Values are the mean±s.e.m. Figure 6: TRP channels agonist-evoked calcium flux responsiveness were impaired in DRG neurons from PN-ZB20KO mice. Primary DRG neurons were isolated from adult control and PN-ZB20KO mice, stimulated with 1 μM capsaicin (TRPV1 agonist), 100 μM MO (TRPA1 agonist) or 250 μM menthol (TRPM8 agonist) and their calcium flux was monitored. ( a ) Capsaicin-responsive neurons were significantly decreased in the DRG from PN-ZB20KO mice. ( b ) Representative traces of Ca 2+ transients evoked by 1 μM capsaicin in DRG neurons of control and PN-ZB20KO mice. A quantity of 80 mM KCl was used to check the viability of the neurons at the end of the experiment. ( c ) The response magnitude was significantly lower in the remaining capsaicin-responsive neurons from PN-ZB20KO DRG than their control counterpart. ( d ) MO-responsive neurons were significantly decreased in the DRG from PN-ZB20KO mice. ( e ) Representative traces of Ca 2+ transients evoked by 100 μM MO in DRG neurons of control and PN-ZB20KO mice. A quantity of 80 mM KCl was used to check the viability of the neurons at the end of the experiment. ( f ) The response magnitude was significantly lower in the remaining MO-responsive neurons from PN-ZB20KO DRG than their control counterpart. ( g ) In neurons from PN-ZB20KO mice, the percentage of menthol-responsive neurons was significantly less than those seen in neurons from control mice. ( h ) Representative traces of Ca 2+ transients evoked by 250 μM menthol in DRG neurons of control and PN-ZB20KO mice. A quantity of 80 mM KCl was used to check the viability of the neurons at the end of the experiment. ( i ) In neurons from PN-ZB20KO mice, the magnitude of remaining responses to menthol was significantly less than those seen in neurons from control mice. The numbers of responsive and total neurons (pooled from all experiments for each genotype) are indicated in ( a , d , j ). ( a , c , d , f , g , i ) Data were analysed by Student’s t -test. ** P <0.01 versus control. Values are the mean±s.e.m. Full size image Decreased currents of TRP channels in PN-ZB20KO DRG Considering TRPV1, TRPA1 and TRPM8 proteins are channels and calcium-imaging data are not sufficient to prove the function of these TRP channels, we further investigated the function of these channels by patch clamp. Whole-cell patch-clamp recordings from acutely dissociated small and medium DRG neurons have been performed in voltage-clamp mode at a holding potential of −70 mV. Typical 1 μM capsaicin-evoked inward TRPV1 currents, 100 μM MO-evoked inward TRPA1 currents and 250 μM menthol-evoked inward TRPM8 currents have been represented as traces in Fig. 7a,c,e . Average TRPV1, TRPA1 and TRPM8 currents densities (pA pF −1 ) have been plotted in Fig. 7b,d,f . A significant decrease in current density was observed in DRG neurons of PN-ZB20KO mice. TRPV1, TRPA1 and TRPM8 currents in DRG neurons significantly decreased from −53.0±3.1 pA pF −1 , −18.1±0.9 pA pF −1 and −14.6±0.8 pA pF −1 in control mice to −22.4±0.7 pA pF −1 ( P <0.01), −6.3±0.6 pA pF −1 ( P <0.01) and −5.2±0.5 pA PF −1 ( P <0.01) in PN-ZB20KO mice, respectively. In other words, TRPV1, TRPA1 and TRPM8 currents in DRG neurons of PN-ZB20KO mice decreased 57.8%, 65.3% and 64.7%, respectively. 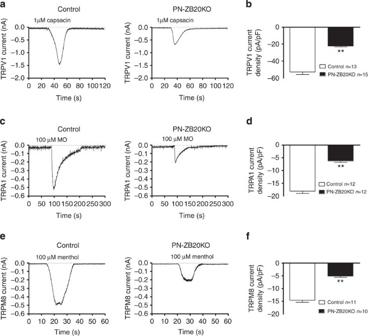Figure 7: Currents of TRP channels were impaired in DRG neurons from PN-ZB20KO mice. (a) Representative traces of TRPV1 current evoked by 1 μM capsaicin in DRG neurons of control and PN-ZB20KO mice. (b) Current density of capsaicin-activated TRPV1 current was significantly decreased in DRG neurons of PN-ZB20KO mice. (c) Representative traces of TRPA1 current evoked by 100 μM MO in DRG neurons of control and PN-ZB20KO mice. (d) Current density of MO-activated TRPA1 current was significantly decreased in DRG neurons of PN-ZB20KO mice. (e) Representative traces of TRPM8 current evoked by 250 μM menthol in DRG neurons of control and PN-ZB20KO mice. (f) Current density of menthol-activated TRPM8 current was significantly decreased in DRG neurons of PN-ZB20KO mice. (b,d,f) Data were analysed by Student’st-test. **P<0.01 versus control. Values are the mean±s.e.m. Figure 7: Currents of TRP channels were impaired in DRG neurons from PN-ZB20KO mice. ( a ) Representative traces of TRPV1 current evoked by 1 μM capsaicin in DRG neurons of control and PN-ZB20KO mice. ( b ) Current density of capsaicin-activated TRPV1 current was significantly decreased in DRG neurons of PN-ZB20KO mice. ( c ) Representative traces of TRPA1 current evoked by 100 μM MO in DRG neurons of control and PN-ZB20KO mice. ( d ) Current density of MO-activated TRPA1 current was significantly decreased in DRG neurons of PN-ZB20KO mice. ( e ) Representative traces of TRPM8 current evoked by 250 μM menthol in DRG neurons of control and PN-ZB20KO mice. ( f ) Current density of menthol-activated TRPM8 current was significantly decreased in DRG neurons of PN-ZB20KO mice. ( b , d , f ) Data were analysed by Student’s t -test. ** P <0.01 versus control. Values are the mean±s.e.m. Full size image Deficient nociception and pain sensation in PN-ZB20KO mice To investigate whether the molecular defects in PN-ZB20KO DRG are accompanied by alterations in behavioural responses to noxious stimuli, we assayed acute responses to thermal and mechanical stimuli, as well as inflammatory pain sensitivity. PN-ZB20KO mice were healthy, fertile and apparently normal. They showed no obvious differences from controls in appearance and spontaneous behaviour. Motor function was tested by rotarod studies and beam walking, and there were no significant differences in the time spent on the rod ( Fig. 8a ) or the number of foot slips on trail of beam walking ( Supplementary Fig. 8 ) between control and PN-ZB20KO mice. 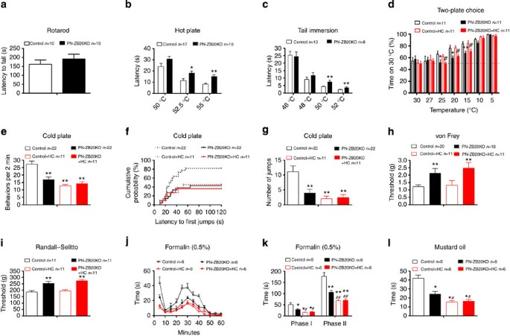Figure 8: Nociceptive behavioural deficits in PN-ZB20KO mice. (a) Rotarod studies showed no motor deficits in PN-ZB20KO mice. (b) Response latencies in the hot plate test. (c) Response latencies in the tail immersion test. (d) In the two-plate choice test, PN-ZB20KO mice showed reduced avoidance of the cooler side when the temperature is between 25 and 15 °C. HC-030031 could not abolish the difference of cold sensation between control and PN-ZB20KO mice. (e) Cold behaviour (number of liftings) was reduced in PN-ZBKO mice in the cold plate test. (f) Cumulative probability plot showing the latency to the first jump off the cold plate in control and PN-ZB20KO mice. (g) Average number of jumps during a 2-min period on a cold plate at 0 °C. HC-030031 significantly alleviated cold-induced nocifensive behaviour of control mice, and abolished the difference of cold sensation between control and PN-ZB20KO mice (e–g). (h) PN-ZB20KO mice showed impaired behavioural response to the mechanical stimulus to the hind paw when using von Frey hairs compared with control mice. (i) PN-ZB20KO mice showed profound analgesia to noxious mechanical pressure when using the Randall–Selitto apparatus compared with control mice. HC-030031 did not affect paw withdraw threshold to mechanical stimulus by von Frey hairs (h) or withdrawal force to noxious mechanical stimulus using Randall–Selitto test (i). (j,k) Time spent licking/biting the injected hind paw in phase I (1–10 min) and phase II (10–60 min) after intraplantar injection of 20 μl of 0.5% formalin was significantly decreased in PN-ZB20KO mice. HC-030031 significantly decreased nociceptive responses and abolished the difference of formalin-induced response between control and PN-ZB20KO mice. (l) Time spent licking/biting the injected hindpaw after intraplantar injection of 20 μl of 0.75% MO was significantly decreased in PN-ZB20KO mice. HC-030031 significantly decreased nociceptive responses and abolished the difference of MO-induced response between control and PN-ZB20KO mice. HC, HC-030031. Data were analysed by Student’st-test (a–c) or analysis of variance followed bypost hoccomparisons (d,e,g–i,k,l). *P<0.05 versus control group; **P<0.01 versus control group; #P<0.05 versus PN-ZB20KO group; ##P<0.01 versus PN-ZB20KO group. Values are the mean±s.e.m. Figure 8: Nociceptive behavioural deficits in PN-ZB20KO mice. ( a ) Rotarod studies showed no motor deficits in PN-ZB20KO mice. ( b ) Response latencies in the hot plate test. ( c ) Response latencies in the tail immersion test. ( d ) In the two-plate choice test, PN-ZB20KO mice showed reduced avoidance of the cooler side when the temperature is between 25 and 15 °C. HC-030031 could not abolish the difference of cold sensation between control and PN-ZB20KO mice. ( e ) Cold behaviour (number of liftings) was reduced in PN-ZBKO mice in the cold plate test. ( f ) Cumulative probability plot showing the latency to the first jump off the cold plate in control and PN-ZB20KO mice. ( g ) Average number of jumps during a 2-min period on a cold plate at 0 °C. HC-030031 significantly alleviated cold-induced nocifensive behaviour of control mice, and abolished the difference of cold sensation between control and PN-ZB20KO mice ( e – g ). ( h ) PN-ZB20KO mice showed impaired behavioural response to the mechanical stimulus to the hind paw when using von Frey hairs compared with control mice. ( i ) PN-ZB20KO mice showed profound analgesia to noxious mechanical pressure when using the Randall–Selitto apparatus compared with control mice. HC-030031 did not affect paw withdraw threshold to mechanical stimulus by von Frey hairs ( h ) or withdrawal force to noxious mechanical stimulus using Randall–Selitto test ( i ). ( j , k ) Time spent licking/biting the injected hind paw in phase I (1–10 min) and phase II (10–60 min) after intraplantar injection of 20 μl of 0.5% formalin was significantly decreased in PN-ZB20KO mice. HC-030031 significantly decreased nociceptive responses and abolished the difference of formalin-induced response between control and PN-ZB20KO mice. ( l ) Time spent licking/biting the injected hindpaw after intraplantar injection of 20 μl of 0.75% MO was significantly decreased in PN-ZB20KO mice. HC-030031 significantly decreased nociceptive responses and abolished the difference of MO-induced response between control and PN-ZB20KO mice. HC, HC-030031. Data were analysed by Student’s t -test ( a – c ) or analysis of variance followed by post hoc comparisons ( d , e , g – i , k , l ). * P <0.05 versus control group; ** P <0.01 versus control group; # P <0.05 versus PN-ZB20KO group; ## P <0.01 versus PN-ZB20KO group. Values are the mean±s.e.m. Full size image In the hot plate, the paw was heated by contact with a hot metal surface. PN-ZB20KO mice had normal withdrawal latencies at temperatures 50 °C, but had significantly longer withdrawal latencies than wild-type littermates at temperatures 52.5 and 55 °C ( Fig. 8b ). Since ZBTB20 is required for nociception in response to thermal stimuli, we inquired whether knock out of ZBTB20 in nervous system resulted in more severe deficiency in the hot plate test. Expectedly, withdrawal latencies of NS-ZB20KO mice were extended further than PN-ZB20KO mice at temperatures 52.5 and 55 °C ( Supplementary Fig. 9 ). In the tail immersion test, the distal portion of the tail was immersed in a heated bath, and the time to tail flick was recorded. PN-ZB20KO mice exhibited normal latencies at <50 °C, but significantly longer response latencies than wild-type mice at temperatures ≥50 °C ( Fig. 8c ). Together, these results show that PN-ZB20KO mice display robust deficits in thermally evoked pain-related behaviour. Given that a previous study showed significant sex-related differences on cold sensitivity [37] , we used male mice in two-plate choice test and cold plate test. Two-plate choice test was used to determine temperature preference of animals or detection of particular temperature ranges [13] . Cold plate (0 °C) test was used to determine nocifensive behaviours response to noxious temperature [11] . In the two-plate choice test, control and PN-ZB20KO mice spent approximately equal time on both plates when both plate surfaces were held at 30 °C ( Fig. 8d ). When the temperature of one plate was reduced, control mice showed a clear preference for the 30 °C side. PN-ZB20KO mice showed reduced avoidance of the cooler side when the temperature is between 25 and 15 °C. However, PN-ZB20KO mice displayed normal preference for 30 °C side when the other side dropped below 15 °C, a demarcation between innocuous cool and noxious cold in primates [38] . These data indicate that the behavioural response to innocuous cold in two-plate choice test is significantly impaired in PN-ZB20KO mice. Considering that both TRPA1 and TRPM8 may be involved in cold sensing, to determine whether TRPA1 is required for in the two-plate choice test, we took advantage of the TRPA1-specific blocker HC-030031. HC-030031 could not alleviate cold-induced behavioural response of control mice ( Fig. 8d ). It is consistent with the results that TRPA1 −/− mice were indistinguishable from control littermates when examined for behavioural responses to cold using the two-plate choice test [13] . These results suggest that TRPA1 does not mediate temperature preference. Furthermore, HC-030031 did not abolish the difference of cold sensation between control and PN-ZB20KO mice ( Fig. 8d ), which suggest the deficit of behavioural response of PN-ZB20KO mice to innocuous cold in two-plate choice test could not result from the deficit of TRPA1. Due to the lack of TRPM8-specific blocker [39] , we could not do similar experiments to address the role of TRPM8 in temperature preference. In the cold plate test, PN-ZB20KO and control mice were placed on a metal cold plate set at a temperature of 0 °C, and their behaviour was observed. PN-ZB20KO mice displayed significantly less nocifensive behaviour (number of liftings) relative to the control mice when left on the cold plate for a 2-min period ( Fig. 8e ). In addition, 81.8% of control mice jumped during 2-min period on the cold plate, suggesting that the cold plate induces significant pain. In contrast, only 40.9% of PN-ZB20KO mice jumped ( Fig. 8f ). Moreover, the total number of jumps was significantly decreased in the PN-ZB20KO mice ( Fig. 8g ). These data indicate that the behavioural response to noxious cold is significantly impaired in PN-ZB20KO mice in the cold plate test. Furthermore, we found HC-030031 significantly alleviated cold-induced nocifensive behaviour of control mice, and abolished the difference of cold sensation between control and PN-ZB20KO mice ( Fig. 8e–g ). These results suggest TRPA1 is critically involved in noxious cold sensing and the defect in cold-evoked nociceptive behaviours of PN-ZB20KO mice in the cold plate test. The response to mechanical stimulation was tested by using von Frey hairs and Randall–Selitto apparatus [40] . As shown in Fig. 8h , PN-ZB20KO mice showed a statistically significant increase of paw withdraw threshold for the von Frey assay. Similarly, application of noxious pressure with Randall–Selitto apparatus revealed a pronounced analgesia in the PN-ZB20KO mice ( Fig. 8i ). TRPA1-specific blocker HC-030031 did not affect paw withdraw threshold to mechanical stimulus by von Frey hairs or tail pressure thresholds to noxious mechanical stimulus using Randall–Selitto test ( Fig. 8h,i ). These results suggest that other molecules than TRPA1 may be involved in the defect in nociception of PN-ZB20KO mice in response to mechanical stimulation. We further investigated inflammatory pain sensation by intraplantar injection of 20 μl of 5% formalin, and the time spent licking or biting the injected hindpaw in phase I (1–10 min) and phase II (10–60 min) was recorded [34] . The first phase is thought to be due to direct chemonociceptive effect of formalin, while the second one is mainly mediated by inflammatory reactions [41] . Surprisingly, PN-ZB20KO mice displayed similar nociceptive responses to 5% formalin as controls ( Supplementary Fig. 10 ). Considering formalin-induced pain behaviours such as licking are positively correlated with formalin concentration [42] , we speculated that 5% formalin might be too high in concentration to produce the behavioural difference between control and PN-ZB20KO mice. Therefore, we used the low concentration of formalin (0.5%) for intraplantar injection as described previously [43] . As expectedly, control mice showed a significant reduction in the first and second phases of the behavioural responses after injection of 20 μl of 0.5% formalin compared with those injected with 20 μl of 5% formalin ( Fig. 8j,k , and Supplementary Fig. 10 ). Importantly, PN-ZB20KO mice displayed an impaired nociceptive response to 0.5% formalin compared with control mice ( Fig. 8j,k ). It is well known that TRPA1 mediates formalin-induced nociception [43] . To further address the role of TRPA1 in the attenuated nociception of PN-ZBKO mice in response to formalin, we used HC-030031 to block TRPA1 before formalin stimulation. Intraperitoneal administration of HC-030031 preceding 0.5% formalin injection significantly decreased nociceptive responses in control and PN-ZB20KO mice, and more importantly, abolished the difference of 0.5% formalin-induced response between these two groups ( Fig. 8j,k ). These results not only support the current notion that TRPA1 is involved in formalin-evoked nociceptive behaviours [43] , but also suggest that decreased TRPA1 expression in nociceptors at least partly explain the defect in formalin-induced inflammatory pain of PN-ZB20KO mice. Moreover, in another model using 20 μl of 0.75% MO solution for intraplantar injection [37] , PN-ZB20KO mice also exhibited a deficit in TRPA1-mediated behavioural responses ( Fig. 8l ). Taken together, these data suggest that ZBTB20 in nociceptors is required for nociception and pain sensation in response to thermal, mechanical and inflammatory stimuli. In this study, we examined the role of ZBTB20 in the primary somatosensory system. Our findings for the first time establish ZBTB20 as a critical regulator of nociception by modulating the expression of a subset of TRP channels in nociceptors. First, ZBTB20 is specifically expressed in the vast majority of nociceptive sensory neurons in DRG. Second, disruption of ZBTB20 decreases the expression of TRPV1, TRPA1 and TRPM8 in DRG neurons, as well as their responsiveness of calcium flux and currents. Third, nociceptor-specific deletion of ZBTB20 results in a marked decrease in the pain sensitivity in response to thermal, mechanical and inflammatory stimuli. Our findings suggest that ZBTB20 plays an essential role in the generation of fully developed nociceptors. Some transcription factors have been identified to regulate nociceptor development. Among them, Ngn1, Brna3 and Klf are critical for the formation and survival of nociceptors during their early development [20] , [22] , [23] , while Runx1 is mainly involved in nociceptor diversification during their later developmental stage [18] , [24] . In addition, Runx1 also regulates the expression of many transduction ion channels and receptors by nociceptors [18] . ZBTB20 expression is initiated in DRG neurons at E13.5, when Runx1 also starts to express. Deletion of ZBTB20 gene either by Nestin-Cre at as early as E11 or by Na v 1.8-Cre at later stage (E14) does not affect the formation, survival or diversification of nociceptors, as evidenced by normal number of small DRG neurons and molecular phenotypes of peripherin, TrkA, c-Ret, CGRP and IB4 in the mutant DRG. Remarkably, nociceptor-specific deletion of ZBTB20 leads to a robust decrease in the expression of TRPV1, TRPA1 and TRPM8. As a result, the corresponding nociceptive sensory neurons, including TRPV1 neurons, TRPA1 neurons and TRPM8 high-positive neurons, are reduced in DRG by the loss of ZBTB20. In contrast to Runx1, ZBTB20 does not affect the expression of sodium channels (Na v 1.7, Na v 1.8, Na v 1.9), ATP-gated channel P2X3, ASIC, Mrgpr members or TRPV2 in DRG neurons. These findings suggest that ZBTB20 is a unique transcription factor regulating the terminal differentiation of a subset of nociceptors. Our findings also suggest that ZBTB20 regulates nociception and pain sensation most likely through modulating the above TRP channels in nociceptors. PN-ZB20KO mice show deficits in pain sensitivity evoked by thermal, mechanical and inflammatory stimulation. TRP channels have been proposed to serve as thermal sensors to temperatures ranging from noxious heat to noxious cold and thus are referred to as thermo-TRPs [4] . Among them, TRPV1 (VR1) and TRPV2 (VRL-1) respond to noxious heat, whereas TRPM8 and TRPA1 are activated by normally innocuous cooling and noxious cold, respectively [4] , [11] . In the present study, we found the expressions of TRPV1, TRPM8 and TRPA1 that are known to be critical in processing pain behaviours in the DRG were decreased in the PN-ZB20KO mice. TRPV1 serve as detectors of thermal stimuli [44] , [45] and mice lacking TRPV1 is impaired in thermal nociception [7] . In the tail immersion test, TRPV1 −/− animals had significantly longer (three- to fourfold) mean withdrawal latencies than wild-type littermates at temperatures greater than 48 °C, but normal latencies at temperatures ≤48 °C. In the hot plate test, TRPV1 −/− mice exhibited normal latencies at 50 °C, but significantly longer response latencies than wild-type mice at temperatures greater than 50 °C. PN-ZB20KO mice, in which TRPV1 is decreased by almost 50%, exhibited an intermediate phenotype consistent with their TRPV1 protein level. Two cold-activated TRP channels have been identified in sensory neurons as transducers of cold stimulation. TRPM8 is activated at temperatures below ~23 °C and chemicals such as menthol and icilin [10] , [12] , while TRPA1 is activated by temperatures below 16 °C and was proposed as a sensor for painful or noxious cold stimuli [17] . Behaviourally, TRPM8 −/− mice cannot discriminate between a warm and a cold surface over a wide range of temperatures that humans consider to be innocuously cool (15–30 °C) or noxiously cold (<15 °C) in the two-plate choice test [13] . In the present study, we found PN-ZB20KO mice showed reduced avoidance of the cooler side when the temperature between 25 and 15 °C, which may be caused by the decreased expression and function of TRPM8 but not TRPA1, since HC-030031 could not abolish the difference of cold sensation between control and PN-ZB20KO mice. It is consistent with the results that TRPA1 −/− mice were indistinguishable from control littermates when examined for behavioural responses to cold using the two-plate choice test [13] , suggesting that TRPA1 does not mediate temperature preference. In the absence of well known and specific blocker of TRPM8 (ref. 39 ), it may not be fully verified that the deficit of temperature preference of PN-ZB20KO mice is resulted from the decreased expression and function of TRPM8, since there may be three general populations of cold-sensitive sensory neurons in DRG: those expressing TRPM8, those expressing TRPA1 and also TRPV1 and those that use neither TRPM8 nor TRPA1 for detecting cold [46] . The role of TRPA1 in noxious cold is still controversial. Some independent studies analysed the effect of TRPA1 deletion on behavioural responses to noxious cold, assessed using cold plate (0 °C) and acetone tests. Kwan et al. and Karashima et al. [11] , [37] found TRPA1 −/− mice showed significantly less nocifensive behaviour than control mice. Bautista et al. [47] , however, found no difference from control. These differences may be explained by difference in methodology, different constructs for TRPA1 deletion and difficulties in assessing cold-induced pain behaviours as described by Foulkes et al. [48] It is worth noting that observation indexes are different in the cold plate (0 ˚C) test. Bautista et al. [47] measured paw-withdrawal latency and time to first shiver, and found responses were not significantly different. Karashima et al. [11] measured number of jumps, percent of mice with jump and latency to first jump and found TRPA1 −/− mice showed significantly less nocifensive behaviour. Conceivably, the phenotype reflects a contribution of TRPA1 to cold sensitivity in the setting of tissue injury, but not to acute cold pain [2] . Furthermore, Karashima et al. [11] did not observe a significant difference in the latency to the first cold-related response such as shivering/paw rubbing, which is consistent with the result of Bautista et al. [47] In the present study, we compared the total number of jumps and percent of mice with jump between control and PN-ZB20KO mice. PN-ZB20KO mice displayed significantly less nocifensive behaviour of jump relative to the control mice. Since HC-030031 significantly alleviated cold-induced nocifensive behaviour of control mice, and abolished the difference of cold sensation between control and PN-ZB20KO mice, we predict that TRPA1 is involved in noxious cold sensing and the defect in cold-evoked nociceptive behaviours of PN-ZB20KO mice in the cold plate test. The role of TRPA1 in mechanosensation is also still controversial. Bautista et al. and Petrus et al. [47] , [49] reported no change in mechanical thresholds in TRPA1 −/− mice, whereas Kwan et al. [37] reported deficits. Whether and how these differential physiological effects manifest at the level of behaviour is unclear [2] . In the present study, TRPA1-specific blocker HC-030031 did not affect mechanical thresholds in control or PN-ZB20KO mice, which suggest that TRPA1 is not involved in mechanosensation in our study and the deficit in nociception of PN-ZB20KO mice in response to mechanical stimulation is not caused by the decreased expression of TRPA1. Combined with the lack of clear evidence of direct mechanical activation of the recombinant mammalian TRPA1 (ref. 50 ), these data raise the possibility that TRPA1 is not intrinsically mechanically sensitive. So far, the molecular basis of mammalian mechanotransduction is far from clarified [2] . Therefore, the exact mechanisms need future study. For example, it is known that hyperpolarizing channels such as the TREK and TRAAK channels of the K2P channel family control pain produced by mechanical stimulation and both heat and cold pain perception in mice by opposing depolarization of the nociceptors [51] . The expression and function of these channels and other molecules such as Na v 1.7 and Ca v 2.2 related with mechanosensation will be investigated in the future study [2] , [34] , [52] . The formalin model is widely used for assessing inflammatory pain and evaluating the effects of analgesic compounds in laboratory animals. Formalin-induced responses in TRPM8-deficient mice at room temperature were similar to that of wild-type mice [14] . The role of TRPV1 in formalin-induced responses is controversial. Some reports show TRPV1 antagonist significantly decreased formalin-induced responses [53] , [54] , but there are some reports indicating that formalin-induced responses in TRPV1-deficient mice were similar to that of wild-type mice [55] , [56] . However, at the behavioural level, pharmacologic blockade or genetic ablation of TRPA1 produced marked attenuation of the characteristic flinching, licking and lifting responses resulting from intraplantar injection of formalin [43] . These results show that TRPA1 is the principal site of formalin’s pain-producing action in vivo . In the present study, PN-ZB20KO mice showed a significant reduction in 0.5% formalin-evoked pain behaviours, and intraperitoneal administration of HC-030031 preceding formalin injection significantly decreased nociceptive responses and abolished the difference of formalin-induced response between control and PN-ZB20KO mice. PN-ZB20KO mice had an intermediate phenotype compared with mice treated with HC-030031, suggesting that there may be a dosage effect in formalin-induced nociceptive responses. At low doses (≤0.5%), formalin interacts directly with the TRPA1 (refs 43 , 57 ). Furthermore, after intraplantar injection of 0.5% formalin, the expression of activating transcription factor 3 (a reliable marker of nerve injury) in DRG was significantly reduced in TRPA1 −/− mice, but higher doses of formalin (2% or 5%) elicited the same activating transcription factor 3 response in WT and TRPA1 −/− mice [58] . These results indicate that in WT mice, high doses of formalin (>0.5%) recruit both TRPA1- and non-TRPA1-expressing DRG neurons [58] . So, we consider it might be better to use low doses of formalin (≤0.5%) in the experiments of formalin-evoked pain behaviours involving TRPA1. Channels or receptors in DRG are generally expressed in a partially overlapping or mutually exclusive fashion. In adult mice, TRPV1 and TRPM8 are distributed in different class neurons of DRG [17] , and TRPA1 is largely restricted to TRPV1-positive neurons [16] . ZBTB20 protein is distributed in the majority of DRG neurons that express TRPV1, TRPA1 or TRPM8, suggesting that ZBTB20 may regulate the expression of these TRP channels in a cell-autonomous manner. It has been reported that the expression of these nociceptive ion channels is absent or significantly decreased in Runx1 −/− mice [18] . In the present study, we found the expression of Runx1 mRNA was not significantly altered, so the exact mechanisms that link ZBTB20 to the expression of these channels remain unknown. In the previous studies, we have identified some direct target genes of ZBTB20, such as alpha-fetoprotein in liver [59] , fructose-1,6,-bisphosphotase 1 in pancreatic β cells [60] and IκBα in macrophages [61] , in which ZBTB20 function as transcriptional repressors. Logically, decrease in expression of ZBTB20 should result in increase of transcription of target genes. However, in the present study, knockout of ZBTB20 results in decreased expression of the TRP channels. We speculate that ZBTB20 may regulate these genes by indirect mechanisms, which was supported by our ChIP results that ZBTB20 did not bind to the promoters of TRPV1 , TRPA1 or TRPM8 genes. In summary, our identification of ZBTB20 as a critical regulator for the three key TRP channels provides insight into the terminal maturation of nociceptive sensory neurons, which will help to unravel the cellular and molecular basis of nociception and pain sensation. Generation of PN-ZB20KO mice The targeted ES cells carrying the ZBTB20 neo-flox allele were injected into C57BL/6 blastocysts to produce chimeric mice, which transmitted the ZBTB20 neo-flox allele to the progeny. The neomycin resistance cassette was removed by breeding with protamine promoter- Cre transgenic mice. We crossed ZBTB20 flox mice with Na v 1.8-Cre mice, which have the capacity to mediate Cre/loxP recombination exclusively in nociceptor [34] , [35] . After repeated crossings, we obtained ZBTB20 mutant mice ( ZBTB20 flox/flox ; Na v 1.8-Cre ), as well as various genotypes of siblings. From the latter, floxed/Cre-negative, non-floxed Cre-positive or wild-type mice were used as littermate controls. We also crossed ZBTB20 flox mice to Nestin-Cre mice [36] to get the nervous system-specific knockout mice. The mice used in this study were 2- to 6-month-old males or females that had been backcrossed to C57BL/6 mice for at least five generations. Throughout the behavioural experiments, observers were blind to the genotype of each individual animal. Animal experiments were conducted in accordance with the guidelines of the Second Military Medical University Animal Ethics Committee. Immunostaining For immunostaining on frozen sections, the embryos were collected in ice-cold phosphate-buffered saline (PBS), fixed in 4% paraformaldehyde in PBS and saturated with 20% sucrose in PBS overnight at 4 °C. For adult mice, after perfusing with 4% paraformaldehyde in PBS, DRG were dissected and collected in 4% paraformaldehyde for 1 h and saturated with 20% sucrose in PBS overnight at 4 °C (ref. 31 ). Cryostat sections of L4-5 DRGs were processed for single- or double- immunofluorescent staining with mouse monoclonal anti-ZBTB20 antibody 9A10 (1:1,000), goat polyclonal anti-peripherin antibody (1:200, Santa Cruz Biotechnology CA, USA), rabbit anti-neurofilament (N200) antibody (1:1,000, Sigma-Aldrich, MO, USA), lectin IB4-biotin (1:1,000, Sigma-Aldrich), goat polyclonal anti-CGRP antibody (1:4,000, Abcam, MA, USA), rabbit anti-Na v 1.8 antibody (1:1,000; Alomone Labs, Jerusalem, Israel),goat polyclonal anti-TRPV1 antibody (1:200, Santa Cruz Biotechnology), rabbit polyclonal anti-TRPA1 antibody (1:2,000, Abcam) and rabbit polyclonal anti-TRPM8 antibody (1:2,000, Abcam). Quantitative RT–PCR DRG was used as source of total RNA. Real-time RT–PCR was performed in a two step reaction. First-strand cDNA was synthesized with a SuperScript III First-Strand Synthesis Kit (Invitrogen), and the second step was performed in a fluorescent temperature cycler (Mastercycler eprealplex; Eppendorf) with SYBR Green and specific primers for ZBTB20. Every plate included 36B4 gene as internal control. Western blot analysis Total proteins of DRG were electrophoretically separated on 4–15% gradient SDS–PAGE gels and transferred onto nitrocellulose membranes. Membranes were probed with the following primary antibodies: mouse monoclonal anti-ZBTB20 antibody 9A10 (1:1,000); rabbit polyclonal anti-TRPA1 antibody (1:200, Abcam); rabbit polyclonal anti-TRPM8 (1:200, Abcam); goat polyclonal anti-TRPV1 (1:200, Santa Cruz Biotechnology); mouse monoclonal anti-α-tubulin antibody (1:8,000, Sigma-Aldrich). Secondary antibodies were either horseradish peroxidase-conjugated anti-rabbit or anti-mouse IgG (1:8,000, Vector Laboratories). Signals were then generated using a Chemiluminescent Detection Kit (ECL Plus; Amersham Pharmacia Biotech) and visualized with a scanner. Six different preparations of control and mutant DRG individually were used for western blot analysis. Expression levels of each protein of interest were normalized to that of α-tubulin. Neuron counts To count the total number of DRG, adult mice were perfused with 1 × PBS followed by 4% paraformaldehyde. The L4 DRG was identified using the ribs and pelvic bone as landmarks. Eight micron continuous sections of L4 DRG were collected and stained using Nissl substance. Neurons were identified by their large round or oval nuclei [62] . The images of every fourth section of L4 DRG were used to count the number of neurons manually. Neuron numbers for whole ganglia were calculated by summing counts from the individual sections and multiplying by 4. To determine the percentages of neurons expressing molecular markers, we prepared adjacent sets of sections from each L4 DRG. In the experiments of in situ hybridization, some sections were probed with different probes and the adjacent set of them was probed with the pan neuronal marker SCG10 to determine the total number of neurons so that percentages can be calculated. The thickness of sections for in situ hybridization is 8 μm. In the experiments of immunostaining, 12–16 DRG sections per animal (four animals of each genotype) were labelled with anti-TRPV1, anti-TRPA1 or anti-TRPM8 antibodies and the adjacent set of them was used for Nissl staining to determine the number of neurons so that percentages can be calculated. The thickness of sections for immunostaining or Nissl staining is 4 μm. Four to seven independent L4 DRG were used for each counting. In situ hybridization After perfusing with 4% paraformaldehyde in PBS, DRG of adult mice were dissected and collected in 4% paraformaldehyde for 1 h and saturated with 20% sucrose in PBS overnight at 4 °C. DRG were embedded in optimal cutting temperature compound and sectioned at 8 μm. The cryostat sections were treated with 10 μg ml −1 Proteinase K for 15 min followed by fixation in 4% formaldehyde for 15 min, and then were acetylated for 10 min in 0.1 M triethanolamine with 0.25% acetic anhydride. Antisense riboprobes labelled with digoxygenin-UTP were transcribed from cDNA clones [18] . After overnight hybridization with riboprobes, cryosections of DRG were detected with anti-digoxygenin (Roche) antibody conjugated to alkaline phosphatase, and developed with nitro blue tetrazolium. ChIP assay DRGs from five normal adult rats were isolated and pooled together. ChIP assays were performed as described with minimal modifications [59] , [63] . Briefly, DRGs were cross-linked and sonicated. The fragmented chromatin lysate was incubated overnight with specific antibodies: acetyl-histone H3 (Millipore), ZBTB20 (9A10) and normal mouse IgG (Upstate). Then Dynabeads Protein G (Invitrogen) were added to the samples and incubated for 1 h at 4 °C. Purified chromatin DNA was subjected to conventional and quantitative PCR with primers for core promoter regions of rat TRPV1 , TRPA1 or TRPM8 genes ( Supplementary Table 1 ), with acetylated histone 3 as positive control and immunoglobulin G as negative control. The data were analysed using the function 2 –ΔΔCt , where ΔΔCT=(Ct[IP]− C t[input]) SA −(Ct[IP]−Ct[input]) NS . SA, specific antibody, NS, non-specific antibody. Three independent ChIPs were performed. Calcium imaging Adult mice were given an overdose of 4% chloral hydrate. DRG were rapidly excised and dissociated with 40 U ml −1 Papain (Worthington) solution in Hank’s BSS without Ca 2+ and Mg 2+ at 37 °C for 20 min, pelleted and resuspended in 4 mg ml −1 collagenase type II (Worthington) for 20 min. Preps were subsequently subjected to mechanical trituration in a DMEM medium (DMEM supplemented with 10% fetal calf serum). Dissociated neurons were centrifuged, resuspended in the DMEM medium, plated on poly- D -lysine-coated glass coverslips and incubated in 5% CO 2 at 37 °C. Calcium imaging was performed 18–24 h after plating. Cultured adult DRG neurons were loaded for 30 min with 5 μM fura-2 in neurobasal medium with 0.02% Pluronic (w/v) and then rinsed for 30 min in modified Hank’s Balanced Salt Solution (HBSS) composed of the following (in mM): 145 NaCl, 5 KCl, 2 CaCl 2 , 1 MgCl 2 , 10 glucose and 10 HEPES. Coverslips with attached cells were then mounted on a recording chamber and [Ca 2+ ] i in DRG neurons was monitored by a fluorescence microscope system. The cells were perfused with HBSS at a flow rate of 2 ml min −1 . Intracellular [Ca 2+ ] i was measured as absorbance ratio at 340 and 380 nm ( F 340/ F 380) (510 nm for emission) and images were captured at a rate of 1 frame per second using a digital CCD camera. Baseline ratios were recorded for 240 s before bath application of 1 μM capsaicin for 10 s, 100 μM MO for 20 s or 250 μM menthol for 10 s to activate TRPV1, TRPA1 and TRPM8 channels, respectively. After a washout period, cells were perfused by HBSS with high potassium (in mM: 70 NaCl, 80 KCl, 2 CaCl 2 , 1 MgCl 2 , 10 glucose and 10 HEPES.) to check the viability of the neurons. Data are presented as changes in fluorescence ratio ( F 340/ F 380) normalized to baseline ratios. Capsaicin and menthol were dissolved in ethanol, and MO was dissolved in dimethyl sulfoxide) before diluted to a final working concentration. All reagents were prepared fresh daily. For each experimental group, neurons from at least three animals were analysed. Electrophysiological measurements Patch electrodes were fabricated from borosilicate glass with a Micropipette Puller Model 97 (Sutter Instrument Company, CA, USA). Its resistance was 2–4 MΩ when the electrode was filled with the pipette solution. The potential of the electrode was adjusted to zero current between the pipette solution and the bath solution immediately before seal formation. After obtaining a gigaseal, a suction pulse was applied to establish the whole-cell mode. Series resistance was electronically compensated by 70–90%. Recordings were sampled at 5 kHz and filtered at 2 kHz. All experiments were performed at room temperature (20–23 °C). Command pulses were delivered and data were acquired with a patch clamp amplifier (EPC-10, HEKA Elektronik Dr Schulze, Pfalz, Germany) controlled by the PULSE software connected to a computer. Currents of small- to medium-sized neurons were recorded in the whole-cell voltage-clamp configuration with fire-polished borosilicate electrodes [7] . The composition of the external solution was (as mM): NaCl 145, KCl 5, CaCl 2 2, MgCl 2 1, Glucose 10, HEPES 10 (pH adjusted to 7.3 with NaOH). The internal solution contained the following (as mM): KCl 140, CaCl 2 1, MgCl 2 2, EGTA 11, HEPES 10, MgATP 2 (pH adjusted to 7.4 with KOH). Holding potential was −70 mV. Capsaicin (1 μM) and menthol (250 μM) were applied for 10 s to activate TRPV1 and TRPM8 channels, respectively. MO (100 μM) was applied for 20 s to activate TRPA1 channels. Current density was calculated as the ratio between the peak current value and the membrane capacitance to normalize the differences in cell size. For each experimental group, neurons from at least three animals were analysed. Behavioural methods Behavioural experiments were conducted with age- and sex-matched PN-ZB20KO mice and control littermates. Rotarod test Each mouse was given an acclimation training session (four trials, 10 min apart) followed 1 h later by two test trials where the mouse was placed on the rotarod with increasing speed from 4 to 40 r.p.m. over 300 s (ref. 64 ). Each mouse received two consecutive trials and the mean latency to fall was recorded. Beam walking Motor coordination and balance of mice were assessed by measuring the ability of the mice to traverse a graded series of narrow beams to reach an enclosed safety platform [65] . The beams consisted of long strips of wood (1 m) with a 28-, 12- or 5-mm square cross-section or a 28, 17 or 11 mm round diameter, and were placed horizontally, 50 cm above the bench surface, with one end mounted on a narrow support and the other end attached to an enclosed box into which the mouse could escape. Mice were allowed up to 60 s to traverse each beam. The latency to traverse each beam and the number of times the hind feet slipped off each beam were recorded. Hot plate test For the hot plate test, mice were placed on a plate with surface temperature maintained at 50, 52.5 or 55 °C, and the latency for the mouse to lick its hindpaw or jump was recorded. Tail immersion test The terminal 3 cm of animal’s tail was immersed in water which temperature maintained at 46, 48, 50 or 52 °C. The nociceptive end-point was characterized by a jerk of the tail. While nociception measurements were being made, the animals were briefly immobilized (25–30 s) by gently wrapping them in the restrainer. Each mouse received two trials under each temperature and the mean latency to jerk of the tail was recorded. Two-plate choice test Animals were placed in a chamber containing identical adjacent platforms with one set to 30 °C and the other adjusted to various temperatures (30, 27, 25, 20, 15, 10 and 5 °C). Mice were free to explore and the total time spent on each surface was recorded over a 5-min period. Cold plate test For the cold plate test, mice were placed on a plate with surface temperature maintained at 0 °C, and the behaviour was recorded by using a digital video camera. Nocifensive behaviour was quantitatively evaluated by counting the number of liftings and jumps during a 2-min period and by analysis of the latency to the first jump. von Frey test Mice were placed in individual plexiglass chambers on a wire mesh and allowed for 1 h. Mechanical sensitivity was evaluated using a series of calibrated von Frey filaments of graded tension. Calibrated von Frey filaments were applied 10 times per paw with enough force to cause buckling of the filament. The withdrawal threshold for von Frey assay was determined as the filament at which the animal withdrew its paw at least five times in ten applications. Randall–Selitto test Tail pressure thresholds were detected by Randall–Selitto test. The tail was gradually compressed until an escape response was elicited (biting the apparatus, vocalization or struggle) [66] . Three tests separated by at least 15 min were performed for each animal, and the mean value of these tests was calculated. Formalin test Mice were given a subcutaneous injection of 20 μl of 5% or 20 μl of 0.5% formalin into the plantar surface of the right paw, and spontaneous pain behaviour was recorded for 60 min in 5 min intervals starting directly after injection of the irritant into the paw [34] , [43] . The time the mouse spent licking or biting the paw during the first (0–10 min) and second phases (10–60 min) of the test was used for statistical comparisons. MO test Mice were given a subcutaneous injection of 20 μl of 0.75% MO into the plantar surface of the right paw, and spontaneous pain behaviour was recorded for 5 min after injection of the irritant into the paw [37] . The time the mouse spent lifting, licking or biting the paw was used for statistical comparisons. In the experiments to evaluate the role of TRPA1 on nociception, the mice received a single intraperitoneal injection of 100 mg kg −1 HC-030031 or vehicle 60 min before testing. Statistical analyses Statistical analyses were carried out using Student’s t -test or analysis of variance followed by post hoc comparisons. Differences were considered significant when P <0.05. Throughout the paper, data are given as mean±s.e.m. How to cite this article : Ren, A.-J. et al. ZBTB20 regulates nociception and pain sensation by modulating TRP channel expression in nociceptive sensory neurons. Nat. Commun. 5:4984 doi: 10.1038/ncomms5984 (2014).